Crystalline silicon core fibres from aluminium core preforms Traditional fibre-optic drawing involves a thermally mediated geometric scaling where both the fibre materials and their relative positions are identical to those found in the fibre preform. To date, all thermally drawn fibres are limited to the preform composition and geometry. Here, we fabricate a metre-long crystalline silicon-core, silica-cladded fibre from a preform that does not contain any elemental silicon. An aluminium rod is inserted into a macroscopic silica tube and then thermally drawn. The aluminium atoms initially in the core reduce the silica, to produce silicon atoms and aluminium oxide molecules. The silicon atoms diffuse into the core, forming a large phase-separated molten silicon domain that is drawn into the crystalline silicon core fibre. The ability to produce crystalline silicon core fibre out of inexpensive aluminium and silica could pave the way for a simple and scalable method of incorporating silicon-based electronics and photonics into fibres. Silicon (Si) and its oxide silica (SiO 2 ) have both played an important role in modern day electronics and communications [1] , [2] , [3] , [4] , [5] , [6] , [7] , [8] , [9] , [10] . In recent years the opportunities for tighter integration between electronics and photonics have led to the emergence of the field of Si photonics where wafer processes are used to combine the best features of both materials [11] , [12] , [13] , [14] . In a mirror effort the advanced demonstrations of incorporating Si into fibres have been explored in electronics and photonics, such as photodetection [15] , fibre battery [16] , fibre solar cell [17] , [18] , electro-optical modulation [19] , material engineering [20] , non-linear optics [21] , [22] , pressurized Si sphere fabrication [23] and so on. Two disparate methods of producing Si-core silica-cladded fibres have been reported, the first relies on the physical flow process and the second on a chemical reaction internal to a pre-fabricated fibre. In the first method, high-purity Si is placed inside a silica preform and drawn down into a silica fibre with a molten Si core [23] , [24] . The second involves the use of high-pressure Si precursor gas (SiH 4 ) to deposit Si inside a pre-fabricated hollow channel fibre via a chemical vapour deposition (CVD) process [25] . The CVD method is more versatile while the thermal drawing approach is more scalable. The placement of disparate materials thermally drawn into close proximity at elevated temperatures presents compelling opportunities for inducing chemical reactions between the constituent materials [26] , [27] , [28] that could in principle provide the versatility of chemical reactions with the scalability of fibre drawing. Results of this approach that we call fibre-draw synthesis to date have been confined to reactions in only very small domains at an interface between materials. In this work, we utilize the redox reaction between aluminium (Al) and silica (SiO 2 ) during fibre drawing to produce a fibre with a different core composition than that of the preform. This occurs through the following reaction: At high drawing temperature, the metallic Al reacts with the cladding material SiO 2 and reduces the Si. The products (Al 2 O 3 and Si) then get phase separated, thus forming a pure Si-core in silica fibre. The reaction, diffusion and the phase separation all take place at an elevated temperature close to the fibre draw temperature. Fibre fabrication and characterization The proposed method centres on a technique so-called preform-to-fibre fabrication by thermally drawing a macroscopic solid-state preform into extended lengths of uniform fibres, as shown in Fig. 1a . The preform consists of one piece of Al wire (3 cm long, 250 μm diameter) placed inside a silica tube (inner diameter 300 μm, outer diameter 600 μm). This assembly is further cladded with two concentric silica tubes (one with 1 mm inner diameter, 6 mm outer diameter, and the other one with 6 mm inner diameter and 12 mm outer diameter), as shown in Fig. 1b . The chamber where the Al wire resides is then pumped to 10 −3 mbar and sealed with silica rods on both ends to prevent Al in contact with air. The preform with the Al core is then heated up to 2,200 °C in Argon atmosphere and pulled into metre-long fibres with the diameters of ~500 μm. During the fibre draw, Al melts and reacts with the surrounding silica cladding, and reduce Si atoms out of silica [29] . Si atoms accumulate during this process and finally occupy the entire core, resulting in a Si-core fibre with silica cladding, as shown in Fig. 1c . 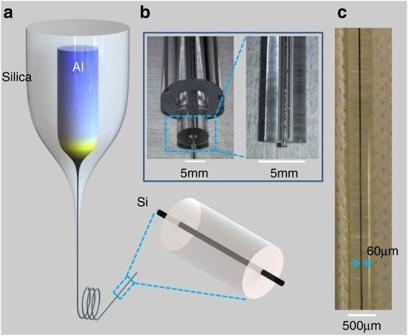Figure 1: Aluminium-core-silica-cladding preform drawn into silicon-core fibre. (a) The schematic diagram of the drawing process. A macroscopic preform with an elemental Al core surrounded with silica is thermally drawn into a fibre with an elemental Si core and a silica cladding. (b) The optical image of the preform before the shiny Al core is sealed in the cladding. (c) The optical image of the drawn fibre with a black Si core. The core diameter is about 60 μm. Figure 1: Aluminium-core-silica-cladding preform drawn into silicon-core fibre. ( a ) The schematic diagram of the drawing process. A macroscopic preform with an elemental Al core surrounded with silica is thermally drawn into a fibre with an elemental Si core and a silica cladding. ( b ) The optical image of the preform before the shiny Al core is sealed in the cladding. ( c ) The optical image of the drawn fibre with a black Si core. The core diameter is about 60 μm. 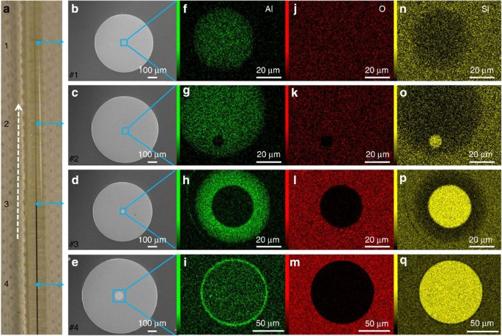Figure 2: Transition of fibre core. (a) The optical image of a piece of fibre where a light-yellow core transits to a black core. The white dashed arrow illustrates the fibre drawing direction. (b–e) The SEM images of the cross-sections at the four labelled locations ina. (f–q) The EDX mappings of the marked area inb–ecorrespondingly. Green, red and yellow denote element aluminium (Al), oxygen (O) and silicon (Si), respectively. Full size image Figure 2a shows an optical image of the fibre and indicates a change in core material as the fibre is drawn. From top to bottom, the colour of the fibre core is seen to transit from light yellow to black. Scanning electron microscope (SEM) and energy-dispersive X-ray spectroscopy (EDX) analyses are taken at four locations along the length of the fibre. Figure 2b–e is SEM images of the cross-sections at locations 1–4 marked in Fig. 2a , respectively. Comparing these four figures, one notice there are light-grey dotswithin the core region in Fig. 2c–e . The grey dot in Fig. 2c is so small that is hardly noticed, but can be seen more clearly from EDX mapping on a zoomed-in area as shown in Fig. 2o . The dots in Fig. 2d,e are much larger. It is worth mentioning though that these dots in Fig. 2c–e , however, are quite different in forming mechanism and in 3D shape. In Fig. 2c the dot is actually a precipitated spherical drop composed of a majority of Si. But in Fig. 2e the dot is actually cross-section of the long crystalline Si wire ( Supplementary Note 1 ). The EDX analyses around these areas are shown to the right of the four SEM images and confirm that the dots in locations #3 and #4 are composed of high-purity Si. In Fig. 2f–q , green, red and yellow colours denote element Al, oxygen (O) and Si, respectively. In Fig. 2f,j,n (location #1), the core is composed mainly of Al and O. In Fig. 2g,k,o (location #2), a small agglomeration of Si appears while Al and O still dominate the core area. In Fig. 2h,l,p (location #3), a large Si core is formed in the centre of the core area, surrounded by a thick layer composed of Al and O. Finally, in Fig. 2i,m,q (location #4 which is in the black core section), Si occupies the entire core region, leaving Al to only a thin layer between the core and the cladding. Figure 2: Transition of fibre core. ( a ) The optical image of a piece of fibre where a light-yellow core transits to a black core. The white dashed arrow illustrates the fibre drawing direction. ( b – e ) The SEM images of the cross-sections at the four labelled locations in a . ( f – q ) The EDX mappings of the marked area in b – e correspondingly. Green, red and yellow denote element aluminium (Al), oxygen (O) and silicon (Si), respectively. Full size image To further explore the differences between the light-yellow and black core regions, transmission electron microscopy (TEM)-based analyses are performed at two different cross-sections (see Supplementary Fig. 1 for preparation of TEM samples), corresponding approximately to locations #2 and #4, respectively. In the core of a yellow-core region, we find that spherical drops form scattered along the axial direction ( Supplementary Fig. 2 ). If we focus on one of these spherical drops, we obtain the results shown in the top panel of Fig. 3 . 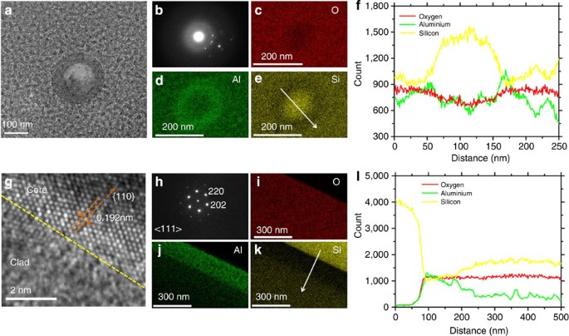Figure 3: Nano-scale analyses on fibre core. On the top panel,a–fdata are measured inside the core region of the fibre with a yellow core (near location #2 inFig. 2a). (a) TEM image, the dot is one of the many dots seen on the sample. (b) The diffraction pattern indicates that the sample is mostly amorphous. (c–e) EDX mappings ona, red, green and yellow denote O, Al and Si, respectively. (f) EDX line scan result. The white arrow ineshows the line scanning path corresponding tof. On the bottom panel,g–ldata are measured at the core-cladding interface of the fibre with a black core (near location #4 inFig. 2a). Ing, the yellow dashed line indicates the interface between the crystalline part (core) and the amorphous part (clad). The parallel orange lines are {110} faces, and the distance between them is measured 0.192 nm. (h) Taken from crystalline side of the yellow line, and the zone axis has been tilted to <111>. (i–k) EDX mappings ong, red, green and yellow denote O, Al and Si, respectively.l, EDX line scan result. The white arrow inkshows the line scanning path corresponding tol. Figure 3a shows that the sphere is about 100 nm in diameter and is surrounded by a circle of different materials. The diffraction pattern in Fig. 3b shows that the materials are mostly amorphous, and the EDX maps in Fig. 3c–e reveal that the sphere is Si rich while the surrounding halo is Al rich. A line scan result across the sphere, as shown in Fig. 3f , confirms this observation. In the case of the black core region (bottom panel), we find distinct properties across the core-cladding interface. As shown in Fig. 3g , the dashed yellow line separates a crystalline part from an amorphous part. Figure 3h is the diffraction pattern taken on the crystalline side and indicates that the material is crystalline with a diamond cubic structure as viewed along <111> zone axis. The two parallel lines highlighted in Fig. 3g represent {110} faces. The distance between the neighbouring faces is 0.192 nm, from which the lattice constant of the crystalline material is calculated to be 0.543 nm. This detailed lattice structure information helps identify that the crystalline material is Si ( Supplementary Fig. 3 , Supplementary Note 2 ). Furthermore, X-ray diffraction (XRD) and Raman spectrum [30] , [31] help identify that the Si core wire is polycrystalline, which is similar to that of the core drawn from molten-core method [18] , [24] ( Supplementary Figs 4 and 5 ). The EDX mappings shown in Fig. 3i–k clearly demonstrate that the thickness of the Al-rich layer surrounding the Si core is about 100 nm. Finally, the line scan in Fig. 3l demonstrates the purity of Si in the core region. Figure 3: Nano-scale analyses on fibre core. On the top panel, a – f data are measured inside the core region of the fibre with a yellow core (near location #2 in Fig. 2a ). ( a ) TEM image, the dot is one of the many dots seen on the sample. ( b ) The diffraction pattern indicates that the sample is mostly amorphous. ( c – e ) EDX mappings on a , red, green and yellow denote O, Al and Si, respectively. ( f ) EDX line scan result. The white arrow in e shows the line scanning path corresponding to f . On the bottom panel, g – l data are measured at the core-cladding interface of the fibre with a black core (near location #4 in Fig. 2a ). In g , the yellow dashed line indicates the interface between the crystalline part (core) and the amorphous part (clad). The parallel orange lines are {110} faces, and the distance between them is measured 0.192 nm. ( h ) Taken from crystalline side of the yellow line, and the zone axis has been tilted to <111>. ( i – k ) EDX mappings on g , red, green and yellow denote O, Al and Si, respectively. l , EDX line scan result. The white arrow in k shows the line scanning path corresponding to l . Full size image Incorporation of crystalline Si into fibres can enable fibre optoelectronic applications. Current approaches include the molten core drawing or high-pressure CVD with post-annealing process, leading to the demonstration of in-fibre semiconductor devices [15] , [17] , [23] , [30] . Here we characterize the electric performance of the Si core fabricated by the fibre-draw synthesis method. As shown in Fig. 4a , 20-nm-thick Al and 150-nm-thick gold (Au) are deposited on selected locations of a piece of Si wire ( Supplementary Figs 6 and 7 , Supplementary Note 3 ). This piece of Si wire is taken from the fibre by etching off cladding with 40% hydrofluoric acid. During the measurement, the 4-point probe method is used to prevent the possible Shottky junction between the Si wire and the electrodes. From Fig. 4b one could get the resistance per unit distance on the Si wire. Because the Si wire is measured to be 100 μm in diameter, the resistivity is calculated to be 0.3 Ω cm (conductivity 3.4 S cm −1 ), which is about the same order as that of the annealed Si core from the high-pressure CVD method and several orders of magnitude smaller than that of intrinsic Si (refs 3 , 30 ). Though exact dopant concentration cannot be obtained through the resistivity value alone, it is highly possible that the Si core is doped instead of intrinsic. Further optimization of structure and fabrication process is supposed to achieve better control of material qualities. 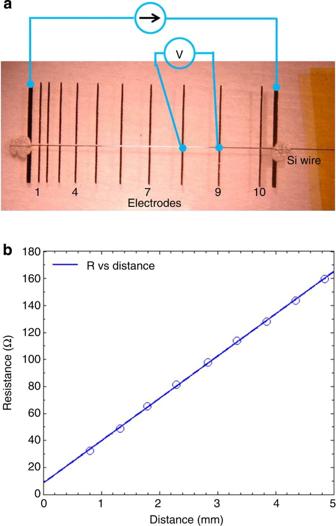Figure 4: Si wire electrical characterization. (a) The 4-point probe measurement set-up. A piece of Si wire (~3 cm long) is taken from fibre by etching off the cladding, and then 20 nm Al and 150 nm Au are deposited on selected locations (2 outmost electrodes for current source and 10 electrodes for voltage metre contact marked 1 to 10). During the measurement, the probe directly contacts the Al/Au layer on top of Si wire. Current is provided from electrodes from two ends, and voltage is measured across neighbourhood electrodes in between the two end electrodes. (b) The resistance across neighbour electrodes are calculated fromaand are plotted against their corresponding distance. Linear regression on the points gives information of Si resistivity. Figure 4: Si wire electrical characterization. ( a ) The 4-point probe measurement set-up. A piece of Si wire (~3 cm long) is taken from fibre by etching off the cladding, and then 20 nm Al and 150 nm Au are deposited on selected locations (2 outmost electrodes for current source and 10 electrodes for voltage metre contact marked 1 to 10). During the measurement, the probe directly contacts the Al/Au layer on top of Si wire. Current is provided from electrodes from two ends, and voltage is measured across neighbourhood electrodes in between the two end electrodes. ( b ) The resistance across neighbour electrodes are calculated from a and are plotted against their corresponding distance. Linear regression on the points gives information of Si resistivity. Full size image Si-core forming mechanism The mechanism for Si material to appear in the fibre is a chemical reaction between the Al core and silica cladding. Al has a melting temperature of 660.32 °C, so it melts when fed into the heating zone and keeps its molten state until oxidized [32] . Also as an active reducer, Al reduces the surrounding silica and produces Si atoms and Al 2 O 3 molecules [33] . The drawing temperature of 2,200 °C is higher than alumina’s melting point so that alumina cannot form a shield to protect Al atoms from oxidizing as it would at room temperature. Without the protection of alumina, the reaction between Al atoms and silica happens very fast due to two factors: (1) as described by Arrhenius’s law, reaction rate relates to temperature exponentially. When the temperature increases by about 2,000 K, the reaction rate is orders of magnitude higher. (2) The largely increased diffusivity at high temperature helps transfer products away from the reaction site at the interface, thus effectively decreasing the products’ local concentration and maintaining the chemical reaction. 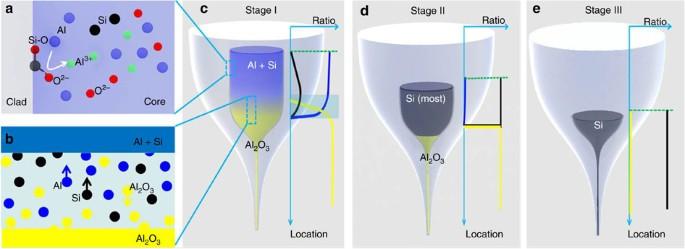Figure 5: Si-core forming mechanism in fibre draw. (a) The chemical reaction at the core-cladding interface. Al atoms (blue) break Si-O bond, reduce Si (black), release O2−ions (red) and change to Al3+ions (green). All the products of ions and atoms dissolve in the Al melt and diffuse into the core. (b) The Si atoms (black), because of their miscibility, diffuse and remain in the Al melt (blue), while ions of O and Al form Al2O3molecules (yellow) and precipitate out at the bottom. (c–e) Sketches of the evolution of the core in the heating zone throughout the drawing process. As the draw continues, more and more Si atoms accumulate in the Al-Si melt and eventually one obtains a highly pure Si melt on top of the Al2O3with all the Al consumed in the redox reaction (Stage II). Further drawing then results in a highly pure Si-core fibre (Stage III). The diagrams corresponding to each figure demonstrate the ratio of different materials along the core axially. Blue, black and yellow denote Al, Si and Al2O3, respectively. The green dashed line that gets lower and lower during the draw marks the position of the core. The cyan shadows inbandcillustrate the location of the transition region. Figure 5a is a schematic depicting how the chemical reaction happens at the core-cladding interface. Figure 5: Si-core forming mechanism in fibre draw. ( a ) The chemical reaction at the core-cladding interface. Al atoms (blue) break Si-O bond, reduce Si (black), release O 2− ions (red) and change to Al 3+ ions (green). All the products of ions and atoms dissolve in the Al melt and diffuse into the core. ( b ) The Si atoms (black), because of their miscibility, diffuse and remain in the Al melt (blue), while ions of O and Al form Al 2 O 3 molecules (yellow) and precipitate out at the bottom. ( c – e ) Sketches of the evolution of the core in the heating zone throughout the drawing process. As the draw continues, more and more Si atoms accumulate in the Al-Si melt and eventually one obtains a highly pure Si melt on top of the Al 2 O 3 with all the Al consumed in the redox reaction (Stage II). Further drawing then results in a highly pure Si-core fibre (Stage III). The diagrams corresponding to each figure demonstrate the ratio of different materials along the core axially. Blue, black and yellow denote Al, Si and Al 2 O 3 , respectively. The green dashed line that gets lower and lower during the draw marks the position of the core. The cyan shadows in b and c illustrate the location of the transition region. Full size image In addition, although the reduced Si atoms are mixed with the other product Al 2 O 3 and not-yet-reacted Al atoms in the beginning, their solubility properties play an important role in separating them and finally forming a Si core. Most importantly, Si is completely miscible with Al in the liquid state, but their solubility with Al 2 O 3 is comparatively low [32] , [34] . As more and more Al 2 O 3 is produced, the excessive Al 2 O 3 precipitates out of molten Al. Meanwhile, Si stays with molten Al because of their miscibility. As the density of molten Al and Si are about 2.4 g cm −3 and are smaller than that of molten alumina that is about 2.8 g cm −3 (refs 34 , 35 , 36 ), molten Al-Si floats up and molten alumina sinks to the bottom as shown in Fig. 5b . As the draw and chemical reaction progress, more and more Al in the Al-Si melt gets consumed hence much less Al 2 O 3 remains in the melt, while Si keeps accumulating in the Al-Si melt on top of alumina melt. Finally, when Al is completely consumed in the reaction, a highly pure Si melt is obtained on the top of the core. Further drawing results in a highly pure Si-core fibre. Figure 5c–e depicts the above-mentioned core composition change during the draw. Solubility not only plays an important role in obtaining a Si-core fibre, but also explains the embedded spheres seen in Fig. 3a as well. Those Si-rich spheres in alumina are from the small amount of Si that dissolves in molten alumina in the heating zone. As the fibre is pulled out of the furnace and the temperature drops, the solubility of Si in Al 2 O 3 decreases. The excess Si then precipitates out and forms spheres in alumina. Besides accumulating with the help of miscibility properties, the Si core is also purified by going through the furnace. Because the preform is fed into the furnace from the top side and the fibre is pulled out of the furnace from the bottom, the difference between the hot furnace temperature and room temperature constructs a temperature profile in which Si melts when entering the hot zone and solidifies when leaving the hot zone. This temperature profile provides the zone melting condition to further purify the Si core [37] . In addition, Si is crystallized when it cools down from liquid state after pulling out of furnace [38] . Our method remains further optimization for future applications. For example, the size of Si-core could be significantly reduced by redesigning the core-clad ratio and adjusting the fibre draw parameters. The redraw technique could also be applied to achieve nanometer-scale Si wires [23] . Also the thin interface layer that lies between the core and the cladding as seen in Figs 2i and 3j could be of interest for the potential advantage on oxygen gettering and surface modification for the post-drawing process [18] , [39] . The smoothness of the Si is verified in the atomic force scan (AFM) image ( Supplementary Fig. 8 , Supplementary Note 3 ). Last but not least, the mechanism of producing Si during fibre drawing is also applicable to other reductive metals, for example, Titanium (Ti) or Calcium (Ca), which could reduce Si because of their more negative reduction potentials [40] . To conclude, we demonstrate a new way to fabricate a high-quality crystalline Si-core fibre by thermally drawing a preform consisting of low-cost metal. The methods described herein set the stage for extending the materials and architecture selections with fibre drawing, thus paving the way towards more sophisticated fibre-based devices. Preform fabrication and fibre drawing For the preform preparation we use the fused-quartz tubes and rods supplied by Technical Glass Products and the Al wire from Alfa Aesar. The fused-quartz capillary fibre (300 μm inner diameter and 600 μm outer diameter) is from Molex Incorporated (product # TSP300794). The coating material on the capillary fibre is burned with flame and cleaned up with isopropanol. The 0.25-mm-diameter Al wire is first inserted into the capillary fibre and then put into a fused-quartz tube with an inner diameter of 1 mm and outer diameter of 6 mm (1 × 6 tube). Two 1-mm-diameter fused-quartz rod are also inserted into the 1 × 6 tube, one on top of the capillary fibre and the other in the bottom of the capillary fibre. The whole assembly is put into a fused-quartz tube with an inner diameter of 6 mm and outer diameter of 12 mm. With the help of propane flame, one end of the structure is fused and the whole assembly is pumped to vacuum and the other end is fused under vacuum. The fibre drawing process starts at the temperature of 2,150 °C and the drawing process continues at 2,200 °C. The preform is fed into the furnace from top with a speed of 1 mm min −1 , and the fibre is pulled out from the bottom end of the furnace with a speed of 660 mm min −1 . The fibre is further coated with coating material, which is called ‘DSM Desotech 3471-3-14(941-314) Desolite single coat coating’, and cured by an in-line ultraviolet coating system. Characterization instruments and methods The SEM images and related EDX mappings on cross-sections of the fibres are taken with the JEOL 6010LA SEM. The TEM samples are prepared in the Helios Nanolab 600 Dual Beam Focused Ion Beam Milling System, and the process of preparing a TEM sample is detailed in the Supplementary Information ( Supplementary Fig. 1 , Supplementary Note 1 ). The TEM images and related EDX scans are taken using the JEOL 2010 FEG Analytical Electron Microscope. The Raman spectrum is taken in the Horiba Jobin Yvon LabRAM Model HR800. The XRD spectrum is taken in Rigaku SmartLab with a parallel-beam optics and capillary-sample set-up. The electrical characterization of the Si wire is on a 4-point stage using the Hewlett-Packard (HP) 4155A Semiconductor Parameter Analyser. The surface smoothness of the Si wire is characterized with Digital Instruments Veeco Dimension 3100 AFM, and the data are processed in the Nanoscope Analysis software (v1.40) from Bruker Corporation. How to cite this article: Hou, C. et al . Crystalline silicon core fibres from aluminium core preforms. Nat. Commun. 6:6248 doi: 10.1038/ncomms7248 (2015).